Symmetrical and asymmetrical division analysis provides evidence for a hierarchy of prostate epithelial cell lineages Although symmetrical and asymmetrical divisions of stem cells have been extensively studied in invertebrate and mammalian neural epithelia, their role remains largely unknown in mammalian non-neural epithelial development, regeneration and tumorigenesis. Here, using basal and luminal cell-specific markers and cell lineage tracing transgenic mice, we report that in developing prostatic epithelia, basal and luminal cells exhibit distinct division modes. While basal cells display both symmetric and asymmetric divisions leading to different cell fates, luminal cells only exhibit symmetrical divisions. Examination of cell division modes in prostate-specific Pten -null mice indicates that both luminal and basal cells can be cellular origins for prostate cancer. Furthermore, analysis of Sox2-expressing cells in p63 and Pten -null mice suggests that basal cells contribute to the luminal population and tumorigenesis. These findings provide direct evidence for the existence of a hierarchy of epithelial cell lineages during prostate development, regeneration and tumorigenesis. The prostate develops from the embryonic urogenital sinus and undergoes rapid ductal morphogenesis postnatally. The adult prostatic epithelium is composed of basal and luminal cells as well as rare neuroendocrine cells. Basal cells express p63, cytokeratin 5 (CK5) and CK14, while luminal cells express CK8, CK18, Nkx3.1 and androgen receptor (AR). The lineage relationship between basal and luminal cells has recently been under heavy debate. Although renal capsule or subcutaneous transplantation experiments support the traditional view that basal cells have the ability to regenerate the prostate gland by repopulating all prostate epithelial lineages [1] , [2] , [3] , [4] , evidence from the rescued explants of p63 -null mice suggest that luminal cells can sustain a prostate structure independently of basal cells [5] . In addition, with transgenic reporter mice, a population of castration-resistant Nkx3.1-expressing luminal cells has been shown to be able to generate not only luminal cells but also other prostatic epithelial lineages [6] . Furthermore, using a lineage-tracing approach, Choi et al. [7] demonstrated that basal and luminal cells in adult mouse prostates are independent self-sustaining lineages during prostate regeneration. However, using the same approach, other groups reported that in addition to unipotent luminal cells, basal cells can act as multipotent stem cells during prostate development or regeneration [8] , [9] , [10] . Verification of the hierarchical nature of epithelial cell lineages in the prostate is critical for understanding the cellular origins of prostate development as well as prostate tumorigenesis. Generally, it is believed that basal cells are likely the cellular origin of prostate cancer [3] , [4] , [10] , [11] . However, it is also known that prostate cancer always displays a remarkable luminal phenotype including the amplification of luminal cells rather than basal cells and overproduction of luminal-derived prostate-specific protein (PSA) [12] , [13] . Therefore, whether or not luminal cells are a cellular origin for prostate cancer remains an important question. Towards this end, Wang et al. [6] have recently shown that transformation of a luminal stem cell population (castration-resistant Nkx3.1) can result in a rapid formation of high-grade prostatic intraepithelial neoplasia (PIN) and carcinoma. Further experiments from Xin and colleagues [7] have demonstrated that specific deletion of the tumour suppressor phosphatase and tensin ( Pten ) homologue in luminal cells can initiate prostate cancer independently of basal cell participation, although basal cells are shown to be able to give rise to tumours as well. Therefore, additional data are required to further understand the mechanisms by which both basal and luminal cells can be the cellular origins for prostate cancer. Symmetrical and asymmetrical divisions are key features of stem cells to expand their numbers, maintain their self-renewal capability and produce differentiated cells [14] , [15] , [16] . Such cell division mode analysis is a classic approach to study cell lineages, cell fate and relationships between stem cells and differentiated daughter cells. An elegant example is the recent study by Lechler and Fuchs [17] demonstrating that asymmetrical divisions of basal stem cells promote notch-dependent epidermal differentiation [18] . During asymmetrical cell divisions, cell polarity molecules such as Par complex (comprising of Par3, Par6 and aPKC) often function as a conserved polarity determinant to regulate spindle orientation and cell fate specification in both invertebrates and vertebrates [19] , [20] , [21] . In addition, accumulating evidence suggests that Par complex works together with PTEN to maintain epithelial polarity and to prevent epithelial tissue from tumorigenesis [22] , [23] , [24] , [25] , [26] . However, the expression patterns of these polarity molecules and the mechanisms by which they influence cell division modes of stem cells and tumorigenesis in the prostate are unknown. In this study, we focus on cell polarity patterns of the prostatic epithelium and cell division modes of prostatic basal and luminal cells. We observe differential expression patterns of the polarity molecules and distinct cell division modes in the basal and luminal compartments. Moreover, by examining transgenic mouse prostates of K14 CreER/RosaRFP (basal cell lineage tracing), p63 −/− (depletion of basal cells) and Prob Cre/ Pten fl/fl (formation of prostate tumours) mice and comparing them to those of the wild type (Wt), we obtain evidence supporting the notion that there is a hierarchy of prostate epithelial cell lineages during prostate development, regeneration and tumorigenesis. Polarization patterns of basal and luminal cells To identify basal and luminal cells in the developing prostate, we immunostained sections collected from postnatal mouse prostates with specific basal (p63 or CK5) and luminal (CK8 or CK18) cell markers. As shown in Supplementary Fig. 1a–d , these markers unequivocally distinguished basal and luminal cell populations within the epithelium surrounded by the basement membrane. An important feature of epithelial cells is that they are polarized. Previous studies have indicated that polarization in stem cells is necessary for asymmetrical divisions [14] , [15] . However, other studies reported that polarization that is associated with tight junctions or adherens junctions promotes symmetrical divisions [27] , [28] , [29] . To determine the polarization patterns of the prostate epithelium, we performed double immunofluorescence of prostate sections with p63, CK8 and antibodies against the polarization molecules Par3 and aPKC. As shown in Fig. 1a–c , the Par3 protein was expressed in both basal and luminal cells but with different patterns. In luminal cells, Par3 was not only seen at the apical end ( Fig. 1a ), but also colocalized with zonula occludens-1 (ZO-1), a tight junction protein ( Fig. 1b ). In contrast, although Par3 and aPKC were also found at the apical end of scattered basal cells ( Fig. 1c,d ), basal cells did not express ZO-1 ( Supplementary Fig. 1e ). In addition, double immunostaining with the adherens junction marker E-cadherin revealed that luminal cells showed both tight and adherens junctions ( Fig.1e ; Supplementary Fig. 1f ). 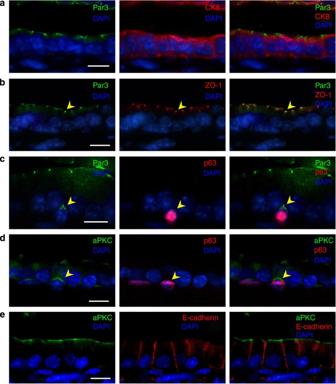Figure 1: Basal and luminal cells exhibit different polarization patterns. (a) Immunostaining of Par3 and CK8 shows that luminal cells are polarized with Par3-dependent tight junctions. (b) Immunostaining of Par3 and ZO-1 shows that Par3 is colocalized with ZO-1 at tight junctions of luminal cells. Yellow arrowheads indicate the tight junctions between two adjacent luminal cells. (c) Immunostaining of Par3 and p63 shows that Par3 is expressed at the apical end in basal cells. Yellow arrowheads point to a basal cell with polarized Par3 location. (d) Immunostaining of aPKC and p63 shows that aPKC is also expressed at the apical end in basal cells. Yellow arrowheads point to a basal cell with polarized aPKC location. (e) Immunostaining of aPKC and E-cadherin shows that prostate luminal cells are connected by tight junctions and adherens junctions, respectively. All sections are originated from anterior lobes of prostate (AP) tissues and counterstained by 4',6-diamidino-2-phenylindole (DAPI) (blue). Scale bars, 10 μm for each related row. Figure 1: Basal and luminal cells exhibit different polarization patterns. ( a ) Immunostaining of Par3 and CK8 shows that luminal cells are polarized with Par3-dependent tight junctions. ( b ) Immunostaining of Par3 and ZO-1 shows that Par3 is colocalized with ZO-1 at tight junctions of luminal cells. Yellow arrowheads indicate the tight junctions between two adjacent luminal cells. ( c ) Immunostaining of Par3 and p63 shows that Par3 is expressed at the apical end in basal cells. Yellow arrowheads point to a basal cell with polarized Par3 location. ( d ) Immunostaining of aPKC and p63 shows that aPKC is also expressed at the apical end in basal cells. Yellow arrowheads point to a basal cell with polarized aPKC location. ( e ) Immunostaining of aPKC and E-cadherin shows that prostate luminal cells are connected by tight junctions and adherens junctions, respectively. All sections are originated from anterior lobes of prostate (AP) tissues and counterstained by 4',6-diamidino-2-phenylindole (DAPI) (blue). Scale bars, 10 μm for each related row. Full size image Basal cells show both symmetrical and asymmetrical divisions The apical localization of polarity proteins may influence the spindle orientation in mitotic cells. Thus, we decided to analyse cell division modes of prostate basal and luminal cells. First, we investigated the spindle orientation of dividing basal cells by staining the sections of developing prostate with CK5 and a marker labelling centrosomes, γ-tubulin. We observed that the mitotic spindles occurred predominantly in two orientations, either vertical or horizontal, relative to the basement membrane ( Fig. 2a ). As cell proliferation was more abundant in the anterior prostate, we mainly focused our analysis in the anterior lobe. At postnatal day 5, ~36% ( n =37/104) of divisions occurred vertically to the basement membrane in the anterior lobe ( Fig. 2b ; Supplementary Table 1 ). As development proceeded, the prostate epithelial lumen became enlarged and the luminal layer was formed. During this process, the vertical divisions increased. At postnatal day 15, ~65% (140/217) of spindles were oriented perpendicularly to the basement membrane ( Fig. 2b ). Similar results were observed in other prostate lobes, including the ventral and dorsolateral lobes ( Fig. 2c ). 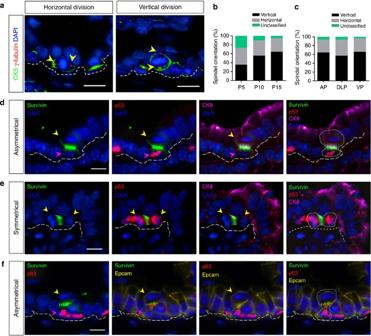Figure 2: Basal cells undergo both symmetrical and asymmetrical divisions. (a) Immunodetection of spindle orientation of a dividing basal cell in metaphase by staining for CK5 and γ-tubulin to indicate either horizontal or vertical divisions. Yellow arrowheads point to the positions of centrosomes indicated by γ-tubulin staining. (b) Quantification of the ratios of horizontal or vertical divisions over the total cell divisions in basal cells during development of anterior prostates. SeeSupplementary Table S1for further data. (c) Quantification of the ratios of horizontal or vertical divisions over the total cell divisions in basal cells in different prostate lobes in P15 mice. SeeSupplementary Table S2for further data. (d) Confocal analysis of cell fate specification in vertical division of basal cells by triple staining for Survivin, p63 and CK8. Yellow arrowheads point to the apical progeny that is p63 negative and CK8 positive, while red arrowheads point to the basal progeny that is p63 positive and CK8 negative. (e) Confocal analysis of cell fate specification in horizontal division of basal cells by triple staining for Survivin, p63 and CK8. Yellow arrowheads point to two daughter cells that are both p63 positive and express low CK8. (f) Immunodetection of asymmetrical division of basal cell by triple staining Survivin, p63 and Epcam. Yellow arrowheads point to the apical progeny that is p63 negative, while red arrowheads point to the basal progeny that is p63 positive. Dashed lines ina,d,e,fdenote the positions of the basement membrane (bold) and the boundary of the dividing basal cells (light). All sections are counterstained by 4',6-diamidino-2-phenylindole (DAPI) (blue). Scale bars, 10 μm for each of the related panels. At postnatal day 15, ~57% ( n =45/79) and 66% ( n =60/91) of basal cells divided vertically to the basement membrane in the dorsolateral prostate and ventral prostate, respectively ( Supplementary Table 2 ). Figure 2: Basal cells undergo both symmetrical and asymmetrical divisions. ( a ) Immunodetection of spindle orientation of a dividing basal cell in metaphase by staining for CK5 and γ-tubulin to indicate either horizontal or vertical divisions. Yellow arrowheads point to the positions of centrosomes indicated by γ-tubulin staining. ( b ) Quantification of the ratios of horizontal or vertical divisions over the total cell divisions in basal cells during development of anterior prostates. See Supplementary Table S1 for further data. ( c ) Quantification of the ratios of horizontal or vertical divisions over the total cell divisions in basal cells in different prostate lobes in P15 mice. See Supplementary Table S2 for further data. ( d ) Confocal analysis of cell fate specification in vertical division of basal cells by triple staining for Survivin, p63 and CK8. Yellow arrowheads point to the apical progeny that is p63 negative and CK8 positive, while red arrowheads point to the basal progeny that is p63 positive and CK8 negative. ( e ) Confocal analysis of cell fate specification in horizontal division of basal cells by triple staining for Survivin, p63 and CK8. Yellow arrowheads point to two daughter cells that are both p63 positive and express low CK8. ( f ) Immunodetection of asymmetrical division of basal cell by triple staining Survivin, p63 and Epcam. Yellow arrowheads point to the apical progeny that is p63 negative, while red arrowheads point to the basal progeny that is p63 positive. Dashed lines in a , d , e , f denote the positions of the basement membrane (bold) and the boundary of the dividing basal cells (light). All sections are counterstained by 4',6-diamidino-2-phenylindole (DAPI) (blue). Scale bars, 10 μm for each of the related panels. Full size image We next investigated the cell fates of the two daughter cells at the anaphase/telophase, as judged by triple staining of the sections with Survivin and cell lineage markers. Survivin is well known as a conserved component of the chromosomal passenger complex, which is localized to the spindle mid-zone in anaphase and concentrates at the mid-body before the abscission of the two sibling daughter cells in telophase [30] . Thus, the subcellular localization of Survivin can effectively indicate the position of two adjacent daughter cells [18] , [31] . Examination of dividing basal cells in late anaphase or telophase revealed that horizontally or vertically aligned daughters cells adopt distinct cell fates, respectively. Although the vertical divisions generated one basal progeny cell and one apical progeny cell that was negative for p63 and positive for luminal marker CK8 ( n =56/58, Fig. 2d ), horizontal divisions of basal cells always gave rise to two basal cells that expressed p63 but not CK8 ( n =36/37, Fig. 2e ). To further confirm whether the two putative cells were indeed two progeny cells during vertical divisions of basal cells, we performed triple staining for Survivin, p63 as well as Epcam, an epithelial cell membrane protein that could clearly highlight the cell boundary during cell divisions. As shown in Fig. 2f , the Survivin staining was unambiguously located at the midline of the two future daughter cells, thus effectively defining the two adjacent cells as sibling cells. Notably, the two progeny cells showed distinct cell fate determinations when the basal cells underwent a vertical division ( Fig. 2f ). Together, these findings indicate that basal cells can undergo either horizontal, symmetrical divisions to give rise to two daughter basal cells or vertical, asymmetrical divisions for a basal and a luminal daughter cell. Luminal cells mainly display symmetrical divisions We next investigated the cell division modes in the luminal compartment and found that there were many dividing cells extending into the prostate lumen, which were negative for the basal cells markers CK5 or p63, but positive for the luminal cell markers CK18 or AR ( Fig. 3a ). In addition, we found that the nuclei of the dividing luminal cells always exhibited apical translocation to the lumen ( Fig. 3a , Supplementary Fig. 2a ). We noticed that such luminal cell division often happened very apically, projected to the lumen, which might be associated with a phenomenon called interkinetic nuclear migration, a classic feature of basal–apical–basal movement during cell division in pseudostratified epithelia [32] , [33] , which was different from dividing basal cells whose nuclei were always close to the basement membrane ( Fig. 2a ). In addition, unlike the dividing basal cells, the spindle orientations of dividing luminal cells were virtually always horizontal to basement membrane at all developmental stages examined ( Fig. 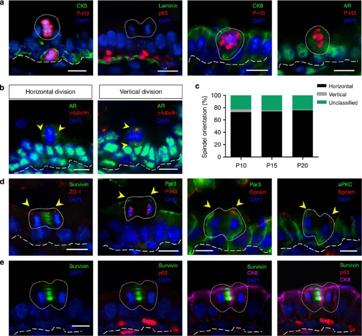Figure 3: Luminal cells mainly exhibit symmetrically horizontal divisions. (a) Immunodetection of dividing luminal cells by staining for CK5 and phosphorylated histone H3 (P-H3, a marker to show the mitotic cell), P63 and laminin, CK8 and P-H3 and AR and P-H3. (b) Defining the spindle orientation of luminal cells by AR and γ-tubulin staining to indicate mitotic spindle orientations of luminal cells, which are either horizontal or vertical to the basement membrane. Yellow arrowheads point to the positions of centrosomes indicated by γ-tubulin staining. (c) Quantification of spindle orientation of luminal cells at different developmental stages of AP prostate lobes (P10, P15 and P20) shows that the spindle orientation of luminal cells is mainly horizontal to the basement membrane. See alsoSupplementary Table S3for further data. (d) Analysis of distribution of polarity proteins in dividing luminal cells by staining for ZO-1 and Survivin, Par3 and P-H3, Par3 and Epcam or aPKC and Epcam. Yellow arrowheads indicate the positions of polarity proteins in dividing luminal cells. (e) Confocal analysis of dividing luminal cells by triple staining for Survivin, p63 and CK8 respectively, indicates that the two daughter cells of horizontal divisions of luminal cells are non-basal, luminal cells. Dashed lines ina,b,d,edenote the positions of the basement membrane (bold) and the boundary of dividing luminal cells (light). All sections are counterstained by 4',6-diamidino-2-phenylindole (DAPI) (blue). Scale bars, 10 μm. 3b, c ; Supplementary Table 3 ), which presumably function to enlarge the lumen during prostate development. 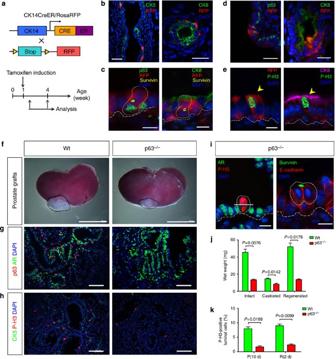Figure 4: Lineage tracing supports the basal to luminal differentiation. (a) Scheme summarizing the genetic strategy used to target RFP expression in K14-expressing basal cells and the protocol used to tracing the fate of basal cells during early prostate development. (b) Immunostaining of CK5 and CK8 with RFP 3 days after tamoxifen injection in newbornK14CreER/RosaRFP mice (1 week). SeeSupplementary Table S7for further data. (c) Immunostaining of p63 and CK8 with RFP 3 weeks after tamoxifen injection in newbornK14CreER/RosaRFP mice. (d) Confocal analysis of cell fates during tolephase of RFP-positive basal cells by staining RFP, Survivin with p63 or CK8. (e) Confocal detection of dividing luminal cell 3 weeks after tamoxifen injection inK14CreER/RosaRFP mice at birth by staining P-H3. Yellow arrowheads point to the dividing RFP+cell that is a CK8-positive luminal cell. (f) Grafts ofp63+/+andp63−/−UGS in renal capsules 10 days post implantation. Dotted lines denote the boundary of prostate grafts. (g) Histological analysis of basal and luminal compartments fromp63+/+andp63−/−grafts stained for AR and p63. (h) Analysis of dividing luminal cells inp63+/+andp63−/−UGS grafts by staining for CK5 and P-H3. (i) Immunodetection of horizontal divisions of luminal cells inp63−/−grafts by staining AR and P-H3, E-cadherin and Survivin. A short line indicates a horizontal spindle orientation. (j) Wet weight ofp63+/+(n=4) andp63−/−(n=3) grafts. (k) Quantification of dividing luminal cells inp63−/−(n=3) andp63+/+(n=3) grafts from histological analysis of P-H3 staining. P10, postnatal day 10; R (2d), androgen replacement was administrated for 2 days from day 14 post castration. Dashed lines ind,e,idenote the positions of the basement membrane (bold) and the boundary of luminal cells (light). Data inj,kare presented as mean±s.e.m., andPvalues were determined by Student’st-test using Prism5. Scale bars, 10 μm (c,e,i), 25 μm (b,d), 50 μm (g) and 100 μm (h), 1 mm (f). Quantitative data from other prostate lobes revealed the same results, that is, dividing luminal cells mainly displayed horizontal divisions relative to the basement membrane ( Supplementary Table 4 ). Examination of polarity complex locations in dividing luminal cells revealed that the Par complex and the ZO-1 tight junction proteins were asymmetrically located at the apical end, but equally distributed into the two daughter luminal cells ( Fig. 3d ; Supplementary Fig. 2b ). Figure 3: Luminal cells mainly exhibit symmetrically horizontal divisions. ( a ) Immunodetection of dividing luminal cells by staining for CK5 and phosphorylated histone H3 (P-H3, a marker to show the mitotic cell), P63 and laminin, CK8 and P-H3 and AR and P-H3. ( b ) Defining the spindle orientation of luminal cells by AR and γ-tubulin staining to indicate mitotic spindle orientations of luminal cells, which are either horizontal or vertical to the basement membrane. Yellow arrowheads point to the positions of centrosomes indicated by γ-tubulin staining. ( c ) Quantification of spindle orientation of luminal cells at different developmental stages of AP prostate lobes (P10, P15 and P20) shows that the spindle orientation of luminal cells is mainly horizontal to the basement membrane. See also Supplementary Table S3 for further data. ( d ) Analysis of distribution of polarity proteins in dividing luminal cells by staining for ZO-1 and Survivin, Par3 and P-H3, Par3 and Epcam or aPKC and Epcam. Yellow arrowheads indicate the positions of polarity proteins in dividing luminal cells. ( e ) Confocal analysis of dividing luminal cells by triple staining for Survivin, p63 and CK8 respectively, indicates that the two daughter cells of horizontal divisions of luminal cells are non-basal, luminal cells. Dashed lines in a , b , d , e denote the positions of the basement membrane (bold) and the boundary of dividing luminal cells (light). All sections are counterstained by 4',6-diamidino-2-phenylindole (DAPI) (blue). Scale bars, 10 μm. Full size image To determine the cell fates of the two sibling cells of dividing luminal cells, we performed triple-immunostaining with antibodies against Survivin, p63 and CK8 and found that the dividing luminal cells did not give rise to any basal cells, but rather always luminal cells ( n =121/121) ( Fig. 3e ). Although more than 70% of divisions of luminal cells exhibited horizontal spindle orientation, the rest of them displayed tilted orientation patterns ( Fig. 3c ). Analysis of the two daughter fates of these non-horizontal dividing luminal cells also showed that they generated only luminal cells that were positive for CK8 ( n =89/89) and did not give rise to basal cells ( n =0/65) ( Supplementary Fig. 3 ). Taken together, in contrast to the dividing basal cells, the dividing luminal cells always underwent symmetrical divisions to produce two luminal daughter cells regardless of the spindle orientations. Prostates re-grow mainly via luminal symmetric divisions To further investigate the division modes of basal and luminal cells in the adult mice, we castrated the adult mice for 3 weeks and then replaced them with androgen for 1 week to induce substantial epithelial cell turnover ( Supplementary Fig. 4a ). Immunohistochemical analyses revealed that both basal and luminal cells proliferated in response to androgen administration; however, luminal cells were obviously more proliferative than basal cells ( Supplementary Fig. 4b ). While ~74% of luminal cells ( n =1299/1755) were positive for Ki67 at 2 days post androgen replacement, only about 6% of basal cells ( n =101/1678) were proliferative, suggesting that luminal cells were more responsive to AR-induced mitogenic signalling and may make a predominant contribution to prostate regeneration due to higher proliferative capability than basal cells. As observed during prostate development, luminal cells always displayed horizontal divisions ( Supplementary Fig. 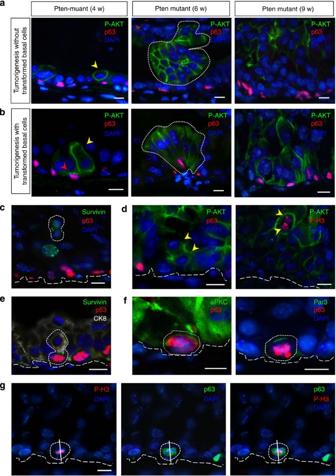Figure 5: Both basal and luminal cells can initiate prostate tumours by different division modes. (a) Immunostaining of APPten-null prostates at different stages (4, 6, 9 weeks) with P-AKT and p63 antibodies indicates a single transformed luminal cell and clones of sole transformed luminal cells. Arrowhead points to a single transformed luminal cell. Dotted lines denote the transformed clone boundary that contains only transformed luminal cells. (b) Immunostaining of APPten-null prostates at different stages (4, 6, 9 weeks) with P-AKT and p63 antibodies indicates a transformed basal cell or mixed clones of transformed basal and luminal cells. Red and yellow arrowheads point to a single transformed basal cell and a single transformed luminal cell, respectively. Dotted lines denote the transformed clone boundary that consists of both transformed luminal cells and basal cells. (c) Division mode analysis of luminal cells by stainingPten-null tumour sections with p63 and Survivin indicates that the transformed luminal cells undergo symmetrical divisions to give rise to daughter cells that are both luminal cells. (d) Division mode analysis of luminal cells by stainingPten-null tumour sections with p63 and P-AKT, or P-H3 and P-AKT antibodies. Arrowheads point to two transformed daughter cells indicated by positive P-AKT staining. (e) Division mode analysis of basal cells inPten-null tumour by staining p63, CK8 with Survivin indicates a dividing basal cell is undergoing asymmetrical division to give rise one basal cell (p63+) and one luminal cell (p63−/CK8+). (f) Cell polarity analysis of basal cells by staining p63 with aPKC, and p63 with Par3. (g) Detection of the dividing basal cells inPten-null prostate by staining P-H3 and p63. Dashed lines denote the cell boundaries or positions of the basement membrane. Scale bars, 10 μm. 4c,e ; Supplementary Table 5 ). However, more than 60% of dividing basal cells showed vertical divisions and about 30% dividing basal cells exhibited horizontal divisions ( Supplementary Fig. 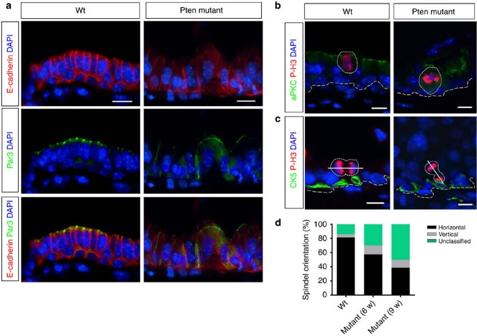Figure 6:Ptenloss disrupts the polarity of luminal cells. (a) Polarity analysis of luminal cells stained for Par3 and E-cadherin in Wt andPten-null prostates (6 weeks). Note thatPtenloss disrupts the polarity of luminal epithelium. (b) aPKC immunostaining of dividing luminal cells in Wt andPten-null prostate sections. (c) Spindle orientation analysis of dividing luminal cells in Wt andPten-mutant prostate by staining for CK5 and P-H3. (d) Quantification of spindle orientations of luminal cells from Wt andPten-null prostate (6, 9 weeks). SeeSupplementary Table S8for further data. Dashed lines inb,cdenote the positions of the basement membrane (bold) and the cell boundary of dividing luminal cells (light). Scale bars, 10 μm for related panels. 4d,f ; Supplementary Table 6 ), suggesting that a higher percentage of asymmetrical divisions occur in regeneration process than that of early development (postnatal day 5 in Fig. 2e ) for a more rapid regeneration of the prostate organ. Further analysis of dividing basal and luminal cells at different regeneration stages revealed that both of them decreased as the regeneration proceeded. Five days post androgen replacement, the regenerated prostate essentially resumed the normal size of an adult mouse prostate, and the proliferation of both basal and luminal cells gradually ceased ( Supplementary Fig. 4b ). Lineage tracing supports the basal to luminal differentiation To provide additional supporting evidence for the asymmetrical division of basal cells to contribute to the luminal lineage, we used basal cell lineage tracing K14 CreER/RosaRFP transgenic mice to trace the fate of K14-expressing basal cells during the early stage of postnatal development ( Fig. 4a ). Tamoxifen administration to newborn K14 CreER/RosaRFP mice induced RFP expression in ~8% of basal cells but not in luminal cells at 3 days post induction ( Fig. 4b ). However, 3 weeks after tamoxifen administration, RFP-expressing cells were observed in both basal and luminal compartments ( Fig. 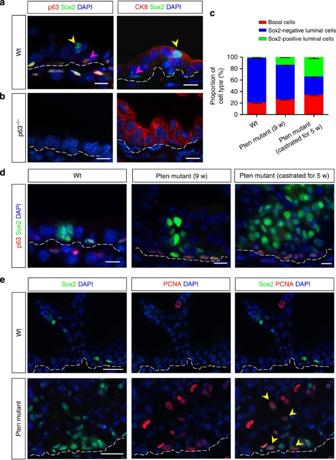Figure 7: Analysis of Sox2+cells in normal andPten-null prostates. (a) Immunostaining of Wt AP prostate lobes with p63, CK8 and Sox2 antibodies. Pink arrowhead points to a basal cell, while yellow arrowhead points to a Sox2-positive luminal cell. (b) Immunostaining of p63-null UGS grafts with p63, CK8 and Sox2 antibodies. Note that no Sox2-expressing luminal cells are detected inp63-null prostates. (c) Quantification of the proportion of basal cells, Sox2-positive luminal cells and Sox2-negative luminal cells from AP lobes of Wt,Pten-mutant (9 weeks) andPten-mutant (castrated for 5 weeks) prostates, respectively. Data are presented as mean±s.e.m. (d) Histological analysis of Sox2-expresing cells in a Wt prostate, aPten-mutant prostate tumour and a castrated prostate tumour stained for Sox2 and p63. (e) Analysis of proliferative status of Sox2-positive cells in Wt, orPten-mutant prostate sections stained for Sox2 and PCNA. Yellow arrowheads point to the double staining cells. Scale bars, 10 μm fora,b,dand 25 μm fore. 4c , Supplementary Table 7 ), suggesting that basal cells have also the differentiating potential to give rise to luminal lineages. To confirm the presence of bi-potent basal progenitors that contribute to luminal cells, we investigated the cell fate during vertical divisions of RFP-expressing basal cells using confocal triple staining for RFP, Survivin and p63 or CK8. We found that the basal cells that carried lineage tracing RFP could divide asymmetrically to generate apical progeny cells that became luminal cells as they were RFP + /p63 − or RFP + /CK8 + ( Fig. 4d ). In addition, we noticed that among all dividing luminal cells at 3 weeks post induction, ~13% (23/177) of them were RFP-positive cells ( Fig. 4e ), suggesting that basal-derived luminal cells can support the expansion of luminal population. Figure 4: Lineage tracing supports the basal to luminal differentiation. ( a ) Scheme summarizing the genetic strategy used to target RFP expression in K14-expressing basal cells and the protocol used to tracing the fate of basal cells during early prostate development. ( b ) Immunostaining of CK5 and CK8 with RFP 3 days after tamoxifen injection in newborn K14 CreER/RosaRFP mice (1 week). See Supplementary Table S7 for further data. ( c ) Immunostaining of p63 and CK8 with RFP 3 weeks after tamoxifen injection in newborn K14 CreER/RosaRFP mice. ( d ) Confocal analysis of cell fates during tolephase of RFP-positive basal cells by staining RFP, Survivin with p63 or CK8. ( e ) Confocal detection of dividing luminal cell 3 weeks after tamoxifen injection in K14 CreER/RosaRFP mice at birth by staining P-H3. Yellow arrowheads point to the dividing RFP + cell that is a CK8-positive luminal cell. ( f ) Grafts of p63 +/+ and p63 −/− UGS in renal capsules 10 days post implantation. Dotted lines denote the boundary of prostate grafts. ( g ) Histological analysis of basal and luminal compartments from p63 +/+ and p63 −/− grafts stained for AR and p63. ( h ) Analysis of dividing luminal cells in p63 +/+ and p63 −/− UGS grafts by staining for CK5 and P-H3. ( i ) Immunodetection of horizontal divisions of luminal cells in p63 −/− grafts by staining AR and P-H3, E-cadherin and Survivin. A short line indicates a horizontal spindle orientation. ( j ) Wet weight of p63 +/+ ( n =4) and p63 −/− ( n =3) grafts. ( k ) Quantification of dividing luminal cells in p63 −/− ( n =3) and p63 +/+ ( n =3) grafts from histological analysis of P-H3 staining. P10, postnatal day 10; R (2d), androgen replacement was administrated for 2 days from day 14 post castration. Dashed lines in d , e , i denote the positions of the basement membrane (bold) and the boundary of luminal cells (light). Data in j , k are presented as mean±s.e.m., and P values were determined by Student’s t- test using Prism5. Scale bars, 10 μm ( c , e , i ), 25 μm ( b , d ), 50 μm ( g ) and 100 μm ( h ), 1 mm ( f ). Full size image To further unveil the prostate epithelial lineage hierarchy and their contributions to development and regeneration, we used the p63 −/− mice, which have been reported to show severe defects in many stratified epithelia [34] , [35] . It has been shown that explants from the p63 -null mice can form prostate glandular structures and undergo several rounds of serial regression/regeneration in the absence of basal cells [5] . Nevertheless, Signoretti et al. [36] have noted that luminal cells can originate from p63-positive basal progenitor cells by complementing p63 −/− blastocysts with p63 +/+ -galactosidase(-gal)-positive ES cells. We isolated urogenital sinuses (UGS) from p63 -null embryos and transplanted them under the renal capsule of male nude mice to investigate cell division modes in the absence of basal cells. We found that although the p63 -null UGS developed ductal structures resembling normal prostate epithelium with lumens, the formed grafts were much smaller than those from transplanted Wt UGS in the renal capsules ( Fig. 4f ). Double immunostaining with a basal cell marker p63 and a luminal cell marker AR indicated that basal cells in the p63 −/− grafts were indeed absent ( Fig. 4g ). Consistent with a previous study [5] , the failure to produce basal cells in the p63 −/− grafts were also confirmed with CK14 and CK5 basal cell marker staining ( Supplementary Fig. 5a ). Examination of ZO-1 and E-cadherin immunostaining showed that tight junctions and adherens junctions were still formed between luminal cells ( Supplementary Fig. 5b ). At different stages of post implantation, quantification of dividing luminal cells (P-H3 positive) showed that the numbers of dividing luminal cells in the p63 −/− grafts were significantly less than that of p63 +/+ grafts ( Fig. 4h ), suggesting that basal cells obviously make an important contribution to the amplification of luminal cells. Further analysis revealed that luminal cells also displayed horizontal, symmetrical divisions to promote the enlargement of prostate lumens ( Fig. 4i ), suggesting that prostate luminal lineage can be self-sustained independently of basal cells. However, the size and wet weight of the p63 −/− prostate grafts were significantly smaller than those of p63 +/+ type ( Fig. 4f,j ). We then castrated the recipient nude mice, and performed androgen replacement to induce regeneration of the prostate. Similar results were obtained, that is, the total number of proliferative luminal cells was remarkably lower than that in the Wt grafts ( Fig. 4k ). Thus, p63-expressing basal cells can also contribute to the dividing luminal cell pool to help enlarge the prostate lumen in a shorter period of time. Cell division mode of transformed luminal cells Next we turned our interest to prostate cancer and investigated the division modes of basal and luminal cells during prostate cancer initiation and progression. As the loss or mutation of the tumour suppressor Pten is known as the most important cause for human prostate cancer, and prostate-specific Pten deletion mouse model ( Prob Cre/ Pten fl/fl ) can recapitulate the entire process of human prostate cancer [37] , we employed this mouse model to capture the mitotic dynamics of basal and luminal cells during prostate cancer initiation and progression. Consistent with previous studies, Pten loss led to an upregulation of the AKT signalling pathway and promoted cell proliferation, as evidenced by the positive staining of P-AKT at the plasma membrane region ( Supplementary Fig. 6a ). Because of this, the cell that is positive for P-AKT is more proliferative and can be regarded as a transformed cell [7] , [38] . To substantiate this point, we performed double immunostaining of the prostate tissue from the Pten -mutant mice with P-APK and proliferation cell nuclear antigen (PCNA). We found that cell proliferation mainly occurred in the P-AKT-positive area ( Supplementary Fig. 6b ). As a negative control, no P-AKT-positive cells were seen in Wt developing or regenerating prostate tissues ( Supplementary Fig. 6a ). Importantly, when P-AKT and p63 double immunostaining was performed with the prostate tissue from Prob Cre/ Pten fl/fl mice, clones of sole transformed luminal cells (PIN lesions) were observed without the participation of transformed basal cells ( Fig. 5a ). At an earlier stage, 6-week-old Pten -mutant prostates, when only small PIN lesions began to form, we detected 31 transformed clones and 20 of them were composed of luminal cells only ( Fig. 5a ). The other 11 clones contained both luminal and basal cells ( Fig. 5b ). As observed during normal prostate development and regeneration, the luminal cells underwent symmetrical divisions to amplify the luminal population during tumorigenesis ( Fig. 5c ). However, unlike the division of normal luminal cells, dividing luminal cells in Pten -mutant prostate display transformed state and can generate transformed progeny luminal cells ( Fig. 5d ). These findings together support the notion that luminal cells can initiate prostate tumours without the participation of basal cells [7] , and that transformation of luminal cells alone will lead to a tumour phenotype that exhibits only amplified luminal cells. Figure 5: Both basal and luminal cells can initiate prostate tumours by different division modes. ( a ) Immunostaining of AP Pten -null prostates at different stages (4, 6, 9 weeks) with P-AKT and p63 antibodies indicates a single transformed luminal cell and clones of sole transformed luminal cells. Arrowhead points to a single transformed luminal cell. Dotted lines denote the transformed clone boundary that contains only transformed luminal cells. ( b ) Immunostaining of AP Pten -null prostates at different stages (4, 6, 9 weeks) with P-AKT and p63 antibodies indicates a transformed basal cell or mixed clones of transformed basal and luminal cells. Red and yellow arrowheads point to a single transformed basal cell and a single transformed luminal cell, respectively. Dotted lines denote the transformed clone boundary that consists of both transformed luminal cells and basal cells. ( c ) Division mode analysis of luminal cells by staining Pten -null tumour sections with p63 and Survivin indicates that the transformed luminal cells undergo symmetrical divisions to give rise to daughter cells that are both luminal cells. ( d ) Division mode analysis of luminal cells by staining Pten -null tumour sections with p63 and P-AKT, or P-H3 and P-AKT antibodies. Arrowheads point to two transformed daughter cells indicated by positive P-AKT staining. ( e ) Division mode analysis of basal cells in Pten -null tumour by staining p63, CK8 with Survivin indicates a dividing basal cell is undergoing asymmetrical division to give rise one basal cell (p63 + ) and one luminal cell (p63 − /CK8 + ). ( f ) Cell polarity analysis of basal cells by staining p63 with aPKC, and p63 with Par3. ( g ) Detection of the dividing basal cells in Pten -null prostate by staining P-H3 and p63. Dashed lines denote the cell boundaries or positions of the basement membrane. Scale bars, 10 μm. Full size image Cell division mode of transformed basal cells We subsequently investigated the division modes of basal cells during prostate tumorigenesis. At 4 weeks, ~5% of basal cells ( n =15/302) in the Pten mutant prostate were transformed as revealed by positive of P-AKT staining, which rose to about 40% ( n =540/1350) at 9 weeks ( Supplementary Fig. 6c ). Compared with that in Wt prostate tissues, Pten loss did not significantly affect the cell fate determination during the vertical division of basal cells, that is, basal cells still underwent asymmetrical divisions to give rise to a daughter luminal cell, which was CK8 + /p63 − and a daughter basal cell, which was P63 + /CK8 − ( Fig. 5e ). Very importantly, in addition to the clone of sole transformed luminal cells, about 34% of clones in the 6-week Pten -mutant mouse were composed of majority of transformed luminal and a small population of transformed basal cells. Among 31 clones of all clustered P-AKT cells, we did not observe the presence of clones composed of sole transformed basal cells. These findings together suggest that transformed basal cells from Pten loss still undergo asymmetrical division to generate luminal progenies that amplify fast and lead to prostate tumours with a luminal phenotype. Pten loss disrupts the polarity of luminal cells Recent studies have revealed that PTEN not only regulates the P-AKT pathway, but also modulates the CDC42-Par signalling pathway, thus participating in the establishment of cell junctions and polarity [39] . Moreover, the PTEN protein itself can bind to the Par complex at tight junctions of epithelial cells [22] , [23] , [24] . Therefore, we examined whether loss of Pten affected cell polarity and spindle orientation of the two types of cells in the prostate tumours of Pten -mutant mice. As shown in Fig. 5f , although Pten loss promoted the proliferation of basal cells by activating AKT pathway, no change in the distribution of polarity molecules was seen in basal cells. About 63% of basal cell ( n =36/57) still underwent vertical divisions ( Fig. 5g ), which showed no significant differences as compared with that in the WT tissue. In contrast to the basal cells, the luminal cells displayed disrupted and reduced polarity (Par3 and aPKC expression patterns) in the transformed luminal cells ( Fig. 6a,b ). In addition, we examined the spindle orientation of these luminal cells. Pten -mutant prostates were collected and sectioned at different developmental stages. Prostate epithelial morphogenesis was normal at 2 weeks, when Cre recombinase did not become activated yet, as shown by negative P-AKT staining ( Supplementary Fig. 6d ). However, by 4 weeks, when Pten became deleted as evidenced by P-Akt staining, the spindle orientation of luminal cells was misoriented with randomly tilted angles ( Fig. 6c,d ; Supplementary Table 8 ). These results suggest that disruption of epithelial polarity due to loss of Pten happens at early stages and may accelerate tumorigenesis. Figure 6: Pten loss disrupts the polarity of luminal cells. ( a ) Polarity analysis of luminal cells stained for Par3 and E-cadherin in Wt and Pten -null prostates (6 weeks). Note that Pten loss disrupts the polarity of luminal epithelium. ( b ) aPKC immunostaining of dividing luminal cells in Wt and Pten -null prostate sections. ( c ) Spindle orientation analysis of dividing luminal cells in Wt and Pten -mutant prostate by staining for CK5 and P-H3. ( d ) Quantification of spindle orientations of luminal cells from Wt and Pten -null prostate (6, 9 weeks). See Supplementary Table S8 for further data. Dashed lines in b , c denote the positions of the basement membrane (bold) and the cell boundary of dividing luminal cells (light). Scale bars, 10 μm for related panels. Full size image Analysis of Sox2 + cells in normal and Pten -null prostates To further investigate the cell lineage relationship during prostate development and tumorigenesis, we focused on the specific prostate stem cell markers as previously reported. We paid particular attention to Sox2 , an important embryonic stem cell transcription factor reported to be a marker of adult stem cells in several types of stratified epithelia [40] , [41] and recently to be associated with castration-resistant human prostate tumour cells [42] , [43] . Immunofluorescence staining revealed that although Sox2 was mainly expressed in basal cells in Wt mice ( Supplementary Fig. 7 ), there were also ~1.6% of luminal cells (141/8695) expressing Sox2 in anterior lobes ( Fig. 7a ). To determine whether or not these small numbers of luminal cells expressing Sox2 were generated from basal lineage, we analysed the renal capsule prostate grafts from p63 -null mice in which basal cells were absent. Interestingly, we did not detect any Sox2-expressing luminal cells in p63 -null prostate grafts ( Fig. 7b ), suggesting that those Sox2-positive luminal cells in Wt prostates are the progeny of basal cells. To determine the potential functions of the Sox2-positive cells during prostate tumorigenesis, we carried out IHC analysis for Pten -mutant tumours. We found that the Sox2-positive luminal cells expanded remarkably during prostate tumorigenesis and became further enriched following androgen deprivation ( Figs 7c,d ). Cell proliferation analysis by PCNA immunostaining showed that while the Sox2-positve luminal cells were negative for PCNA in the Wt prostate, many of them were positive for PCNA in the Pten- mutant prostates ( Fig.7e ), suggesting that Pten loss significantly promoted the proliferation of Sox2 + population. Together, these data suggest that basal cells can give rise to Sox2 + luminal cells and the latter are enriched in prostate tumours. Figure 7: Analysis of Sox2 + cells in normal and Pten -null prostates. ( a ) Immunostaining of Wt AP prostate lobes with p63, CK8 and Sox2 antibodies. Pink arrowhead points to a basal cell, while yellow arrowhead points to a Sox2-positive luminal cell. ( b ) Immunostaining of p63-null UGS grafts with p63, CK8 and Sox2 antibodies. Note that no Sox2-expressing luminal cells are detected in p63 -null prostates. ( c ) Quantification of the proportion of basal cells, Sox2-positive luminal cells and Sox2-negative luminal cells from AP lobes of Wt, Pten -mutant (9 weeks) and Pten -mutant (castrated for 5 weeks) prostates, respectively. Data are presented as mean±s.e.m. ( d ) Histological analysis of Sox2-expresing cells in a Wt prostate, a Pten -mutant prostate tumour and a castrated prostate tumour stained for Sox2 and p63. ( e ) Analysis of proliferative status of Sox2-positive cells in Wt, or Pten -mutant prostate sections stained for Sox2 and PCNA. Yellow arrowheads point to the double staining cells. Scale bars, 10 μm for a , b , d and 25 μm for e . Full size image Although recent studies using genetic mouse models suggest that there are different types of prostate stem cells, demonstration of a hierarchy of cell lineages and cell fate specification of stem cells requires evidence from analysis of symmetrical and asymmetrical division [18] , [21] . The present study demonstrates that the prostatic basal and luminal cells exhibit different division modes. While basal cells display both symmetric and asymmetric divisions leading to different cell fates, luminal cells only exhibit symmetrical divisions producing two luminal cells. For basal cells, they can undergo either symmetrical divisions to produce two daughter basal cells or asymmetrical division to generate one basal cell and one luminal cell. The former occurs with high frequency during early development and adult regeneration, whereas the latter happens increasingly during late development and adult regeneration. Luminal cells, in contrast, only display symmetrical divisions to generate two luminal cells and do not have the capacity to produce any basal cells. The asymmetrical division of basal cells is unambiguously demonstrated not only by triple labelling with both basal and luminal markers at the same time, but also by using basal cell lineage-tracing mice. Consistent with our results, such different cell division modes have been observed in neuroepithelial cells and neuroblasts of Drosophila in which neuroblasts undergo asymmetrical divisions with a parallel spindle orientation to the apical–basal axis, while neuroepithelial cells divide symmetrically, perpendicular to the apical–basal axis [44] , [45] . By cell division mode analysis, our findings strongly support the model proposed recently by Ousset et al . [8] that there is a hierarchy of epithelial lineages containing multi- and unipotent stem cells in the developing prostate. Because accumulating evidence suggests that cancer cells may arise from transformed normal stem cells [46] , [47] , demonstration of the existence of hierarchical stem cells in the normal prostate epithelium would be important for understanding the cellular origins of prostate cancer. Over the past several years, different studies have provided evidence for different cellular origins for prostate cancer [7] , [11] . On the other hand, one important feature of prostate cancer is that this disease always displays luminal phenotypes and basal cell carcinoma is very rare. The present study provides an explanation for these phenomena ( Supplementary Fig. S8a ). While the transformed luminal cells can initiate prostate tumours independently of basal cells via symmetrical divisions, the transformed basal cells appear to produce prostate tumours via expansion of the transformed daughter luminal cells derived from asymmetrical divisions ( Supplementary Fig. S8a ). The latter would then behave just like the transformed luminal cells by symmetrical divisions. In this way, a mixed clone of a small number of basal cells with a much larger number of luminal cells within the PIN lesions are seen ( Fig. 5 ). Similar results are reported by Tang and co-workers [48] , showing that PSA + prostate cancer cells (luminal-like cells) undergo exclusive and more rapid, symmetrical cell divisions to generate more PSA + cells, whereas a faction of PSA −/lo cells (ALDH + CD44 + α2β1 + phenotype, basal-like cells) undergo asymmetric cell divisions. These findings together are essentially in agreement with a recent lineage-tracing study proposing that basal cells need to differentiate into transformation-competent luminal cells and then initiate prostate cancer [7] . On the other hand, it should be pointed out that even though Prob Cre/ Pten fl/fl mouse line is a widely used prostate cancer model, it has some limitation due to its non-exclusive transformation in luminal and basal cells. It would be interesting to compare the cell division modes in CK14 CreER/ Pten fl/fl or CK8 CreER/ Pten fl/fl with Prob Cre/ Pten fl/fl mice in the future. Cell polarity is one important feature of the epithelium [49] and has been shown to affect cell division modes [14] , [27] and tumorigenesis [50] , [51] . Our study indicates that the different expression patterns of the Par3 protein are observed in luminal and basal cells ( Supplementary Fig. S8b ). In luminal cells, Par3 is colocalized with ZO-1 at the apical region to establish tight junctions and has been reported to promote horizontal spindle orientation. In addition, recently studies have suggested that the Par complex may help to maintain the integrity of apical–basal polarity by promoting the establishment of adherens junctions. The latter have been shown to promote the horizontal, symmetrical division of epithelial cells [28] . In sharp contrast, the Par complex in basal cells does not colocalize with ZO-1 to form tight junctions and this might be a reason why the basal cells can have a vertical spindle orientation and undergo asymmetrical divisions. On the other hand, emerging evidence suggest that mutations of Par complex members are intricately related to advanced stages of tumour progression and invasiveness [25] , [26] . In fact, a previous study has revealed a direct association of Par3 with PTEN and that loss of Pten prevents normal development of the apical surface and lumen [22] , [39] . Consistent with these results, our analysis of prostate tumours in the Pten -mutant mice indicates that Pten loss significantly affects the polarity of luminal cells by disrupting the apical location of the Par3 complex at tight junctions. As a consequence of the loss of polarity, the spindle orientation of dividing luminal cells becomes random, which appears to lead to disorganization of the prostate acinar structures and accelerates PIN lesion formation. However, the polarity of basal cells appears unchanged after Pten loss, and thus, the spindle orientation and cell fate specification of basal cells are unaffected. This may explain why the transformed basal cells still have the capacity to undergo asymmetrical divisions to generate transformed luminal cells, which are likely the cells that in turn generate prostate tumours displaying a luminal cell phenotype. Clearly, more studies are needed to demonstrate an outcome of basal or luminal compartment in the Par complex-mutant mice and to determine whether division modes of both basal and luminal cells, the hierarchy of prostate epithelial lineages and basal vesus luminal cell composition within the tumours are affected by the loss of Par complex. It is interesting to note that our analysis of stem cell marker Sox2 demonstrates that Sox2 is expressed in the vast majority of basal cells and a small population of luminal cells in Wt mouse prostates. However, in the p63 -null mutant mice where all basal cells are absent, Sox2-positive luminal population is no longer seen ( Fig. 7 ). This observation reinforces the idea that the basal cells are able to give rise to luminal cells. Interestingly, in Pten -null mutant prostates, these Sox2-expressing luminal cells are more proliferative, remarkably expanded and become even more enriched following androgen deprivation ( Fig. 7 ). As recent studies in several stratified epithelia have shown that Sox2-expressing cells can serve as adult stem cells that play a critical role in the epithelial tissue homeostasis and turnover [40] , our findings implicate that the Sox2-expressing basal cells likely act as stem cells and may contribute to prostate development and regeneration by producing Sox2-expressing luminal cells. However, once transformed by oncogenic mutation such as Pten deletion, they may possibly act as cancer stem cell-like cells that presumably make more important contributions than those Sox2-negative cells to promote the initiation and progression of prostate cancer. Additional supporting evidence for this notion come from previous studies reporting that Sox2-expressing human prostate cancer cells have higher tumorigenic capability [43] , and are more castration resistant [42] . Future studies using Sox2 promoter–reporter in couple with FACS sorting approaches will shed additional light on our understanding of cell division modes, cell fate determination and prostate tumorigenesis. Experimental animals In addition to Balb/c mice, p63 -null, RoasRFP, Prob Cre, Pten fl/fl mice were introduced from Jackson laboratory. K14 CreER transgenic mice were obtained from Model Animal Research Center of Nanjing University. All mice were maintained and used in compliance with the ethical regulations at Renji Hospital. The animal protocols were approved by the Renji Hospital Laboratory Animal Use and Care Committee. Prostates of male mice were collected for histology and immunostaining. Castration and androgen replacement To investigate the cell division modes during prostate regeneration, male Balb/c and nude mice were castrated. At 3 weeks post castration, testosterone pellets (15 mg per pellet per mouse) were implanted subcutaneously. At different regeneration stages, prostates tissue or explants were collected for next immunoassaying analysis. To investigate the cell division modes during prostate cancer, male Pten -null mouse (2, 4, 6, 9 weeks) prostates were collected for immunofluorescence analysis. To investigate the cell division modes in the absence of basal cells, UGS from p63 −/− and p63 +/+ embryos were implanted under the renal capsule of male nude mice. Fourteen days post implantation, nude mice were castrated and supplemented with androgen to examine cell proliferation of p63 −/− and p63 +/+ grafts during regeneration. At different stage of post implantation (10 days, 20 days) or regeneration (2 days), grafts were collected and sectioned for immunofluorescence analysis. Cell lineage tracing For tracing the fates of basal cells, K14 CreER/RosaRFP newborn mice were induced with 1 mg tamoxifen (20 mg ml −1 solution; Sigma). Tamoxifen was dissolved into corn oil and administrated by intraperitoneal injection into experimental mice at the age of 1 week. After tamoxifen induction of 3 days and 3 weeks, prostate sections were analysed by immunofluorescence staining for RFP, CK5, CK8, p63. For detecting the fates of dividing basal cells, confocal analysis was performed to detect the anaphase/telophase cells by triple staining for the spindle mid-body marker Survivin combined with cell lineage markers p63 and CK8. Immunofluorescence Frozen sections were cut at a thickness of 8 mm and fixed in 4% paraformaldehyde in phosphate-buffered saline (PBS) for 30 min. The sections were washed with PBS and transferred to a blocking solution (10% PBS containing 1% normal goat serum) for 1 h at room temperature. After blocking, specimens were incubated with the primary antibodies diluted in PBS containing 1% normal goat serum for overnight at 4 °C. Primary antibodies were rinsed twice in PBS and washed twice for at least 15 min each before the addition of the secondary antibodies for 30 min at room temperature. After washing twice in PBS for at least 15 min each, secondary antibodies, conjugated to Alexa-488, 594 or Cyanine-Cy3 (Jackson Laboratories), were added for 1 h at room temperature. Secondary antibody was rinsed and washed with PBS twice before being mounted on slides with Vector Shield mounting medium containing DAPI (Vector Laboratories). The following primary antibodies were used: mouse anti-p63 (1:100, Santa Cruz, sc-8431), rabbit anti-CK5 (1:500, Epitomics, 1988-1), mouse anti-CK8 (1:500, Covance, MMS-162 P), rabbit anti-CK8 (1:500, Epitomics,2032-1), rabbit anti-CK18 (1:500, Epitomics, 3258-1), mouse anti-E-cadherin (1:300, BD, 610181), rabbit anti-E-cadherin (1:500, Epitomics, 1702-1), rabbit anti-P-AKT (1:500, Cell Signaling, 3787), rabbit anti-Survivin (1:500, Cell Signaling, 2808), rabbit anti-Par3 (1:300, Millipore, 07-330), rabbit anti-aPKC (1:200, Santa Cruz, sc-216), mouse anti-γ-tubulin (1:500, Sigma, T6557), mouse anti-ZO-1 (1:300, Invitrogen, 339100), rabbit anti-Ki67 (1:500, Epitomics, 2746-1), mouse anti-P-H3 (1:500, Cell Signaling, 9706 ), mouse anti-PCNA (1:500, Cell Signaling, 2586), rabbit anti-AR (1:500, Epitomics, 3165), rabbit anti-Laminin (1:500, Abcam, ab11575) and rabbit anti-Sox2 (1:500, Epitomics, 2683-1), rabbit anti-Epcam (1:200, Epitomics, 1144-1), mouse anti-Epcam (1:100, Santa Cruz, sc-66020), rabbit anti-RFP (1:100, MBL, PM005), goat anti-Survivin (1:50, Santa Cruz, sc-8807 ), rat anti-CK8 (1:300, DSHB, TROMA-1). Quantitative analysis of spindle orientation and cell fate Prostate sections were stained with γ-tubulin, Survivin or P-H3 and in a combination with CK5 to distinguish basal cells from luminal cells. Because dividing luminal cells always displayed a nuclear translocation to the apical surface whereas dividing basal cells did not do so, it was easy to distinguish dividing luminal cells from dividing basal cells. Spindle angles of basal or luminal cells in late metaphase or anaphase were determined by division planes, which are shown by centrosome staining to the basement membrane reference line. Division planes positioned at 60–90 degrees to the basement membrane were classified as vertical divisions, and those that were oriented at 0–30 degrees were classified as horizontal divisions. For cell fate analysis, prostate sections were triple stained with Survivin and cell lineage markers p63 and CK8. As Survivin was present at the mid-zone between two daughter cells’ nuclei during anaphase and telophase, we could distinguish definitively the fate specification of two daughter cells. If two daughter cells both expressed p63, we defined it as symmetrical division of a given basal cell. If one daughter cell expressed p63 but the other failed to do so and become CK8 positive, we defined it as asymmetrical division of a basal cell. In contrast, luminal cells always underwent horizontal, symmetrical divisions to generate only luminal cells and did not give rise to basal cells. The ratios of vertical and horizontal divisions of basal or luminal cells are described in Supplementary Tables . Microscopic image acquisition and statistical analyses Sections processed for immunofluorescence staining were analysed under a Leica DM2500 fluorescence microscope equipped with a Leica DFC420c camera and a LAS V3.8 software. Triple-immunofluorescence staining was analysed by confocal laser scanning microscopy (Leica SP5 II, Germany). Images were merged or displayed using the ImageJ software. All data are presented as mean±s.e.m. Data were analysed by Student’s t -test for comparisons between two groups using Prism5. How to cite this article : Wang, J. et al. Symmetrical and asymmetrical division analysis provides evidence for a hierarchy of prostate epithelial cell lineages. Nat. Commun. 5:4758 doi: 10.1038/ncomms5758 (2014).